An ultrafast nickel–iron battery from strongly coupled inorganic nanoparticle/nanocarbon hybrid materials Ultrafast rechargeable batteries made from low-cost and abundant electrode materials operating in safe aqueous electrolytes could be attractive for electrochemical energy storage. If both high specific power and energy are achieved, such batteries would be useful for power quality applications such as to assist propelling electric vehicles that require fast acceleration and intense braking. Here we develop a new type of Ni–Fe battery by employing novel inorganic nanoparticle/graphitic nanocarbon (carbon nanotubes and graphene) hybrid materials as electrode materials. We successfully increase the charging and discharging rates by nearly 1,000-fold over traditional Ni–Fe batteries while attaining high energy density. The ultrafast Ni–Fe battery can be charged in ~2 min and discharged within 30 s to deliver a specific energy of 120 Wh kg −1 and a specific power of 15 kW kg −1 . These features suggest a new generation of Ni–Fe batteries as novel devices for electrochemical energy storage. Using electricity, instead of internal combustion engines, to propel vehicles is an effective way of reducing greenhouse gas emission and consumption of non-renewable fossil fuels. Thus far, batteries have been considered the most suitable devices for powering hybrid electric vehicles and all-electric vehicles [1] , [2] , [3] , [4] , [5] . To meet the challenges facing battery powered vehicles, it is necessary to significantly increase the specific power output and energy capacity of batteries. It is also important to lower the cost and meet the stringent safety requirements of batteries for all-electric vehicles. These characteristics are also important for batteries in storing energy from electrical grids supported by intermittent energy sources such as solar, wind and hydropower. Although Li ion batteries are of high efficiency and energy density, they are expensive and could be unsafe because of the flammability of organic electrolytes and high reactivity of Li containing electrode materials [6] , [7] , [8] . It is worthwhile exploring other battery systems that could operate with materials of low cost in safe aqueous electrolytes. The nickel–iron battery was invented by Waldemar Jungner and Thomas Edison in 1899–1902 and fully developed over the past century [9] , [10] . With NiO(OH) as the cathode and Fe as the anode, a typical Ni–Fe battery is able to deliver specific gravimetric energy of ~30–50 Wh kg −1 and power of ~3–50 W kg −1 (refs 9 , 10 ). With a long cycle life even under harsh conditions, the Ni–Fe battery is known to be a robust and durable power source that has been used for a long time [10] . Importantly, both Ni and Fe are abundant elements on earth and relatively nontoxic. Other than the drawback of low power and energy density relative to Li ion batteries, Ni–Fe battery is highly desirable for renewable energy storage. It is interesting to revisit the century-old Ni–Fe battery and address whether it is possible to significantly improve the specific capacity of Ni–Fe batteries at high charging and discharging rates, aimed at modern hybrid electric vehicle and all-electric vehicle applications, such as to assist Li ion batteries during acceleration and regenerate braking energy, and grid applications such as load following and frequency regulation where fast response is needed. Here we report a new generation of high-performance rechargeable ultrafast Ni–Fe battery (ultra-Ni–Fe battery) capable of ultrafast operations for both charging and discharging enabled by using inorganic/carbon hybrid electrode materials, including Ni(OH) 2 nanoplates grown on oxidized multi-wall carbon nanotubes (MWNTs) as the cathode and FeO x nanoparticles grown on reduced graphene oxide (GO) sheets as the anode ( Fig. 1 ). Direct growth of electrochemically active inorganic nanomaterials on mildly oxidized nanocarbon materials affords desirable morphology, size and dispersion of the active materials [11] , [12] , [13] . It also allows for strong covalent coupling between inorganic nanocrystals and carbon, leading to rapid electron transfer from active materials to current collectors [12] , [14] , [15] , [16] . Charged in ~2 min and discharged in less than 30 s, our ultra-Ni–Fe cell based on such hybrid materials delivers a specific capacity of 115 mAh g −1 based on the mass of the active materials, corresponding to an energy density >120 Wh kg −1 and a power density >15 kW kg −1 . The rate capability of the ultra-Fe–Ni battery is higher than that of conventional Ni–Fe batteries by nearly 1,000 times. At a high current density of 37 A g −1 , the coulombic efficiency of our ultra-Ni–Fe cell is nearly 100%. The charge–discharge cycling stability of our battery currently shows an ~20% capacity decay over 800 cycles, which is an aspect requiring further improvement. 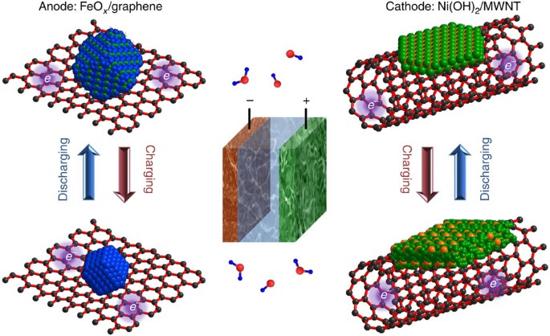Figure 1: Schematic drawing of the ultra-Ni–Fe battery made from inorganic/carbon hybrid materials. A Ni(OH)2/MWNT hybrid was used as the cathode and a FeOx/graphene hybrid was used as the anode. 1 M aqueous KOH solution was used as the electrolyte. On charging, Ni(OH)2/MWNT and FeOx/graphene were converted to NiOOH/MWNT and Fe/graphene, respectively. On discharging, NiOOH/MWNT and Fe/graphene were converted back to Ni(OH)2/MWNT and FeOx/graphene, respectively. Figure 1: Schematic drawing of the ultra-Ni–Fe battery made from inorganic/carbon hybrid materials. A Ni(OH) 2 /MWNT hybrid was used as the cathode and a FeO x /graphene hybrid was used as the anode. 1 M aqueous KOH solution was used as the electrolyte. On charging, Ni(OH) 2 /MWNT and FeO x /graphene were converted to NiOOH/MWNT and Fe/graphene, respectively. On discharging, NiOOH/MWNT and Fe/graphene were converted back to Ni(OH) 2 /MWNT and FeO x /graphene, respectively. Full size image Ni(OH) 2 /MWNT hybrid as cathode for ultra-Fe–Ni battery The cathode of our ultra-Ni–Fe battery was consisted of a Ni(OH) 2 /MWNT hybrid material, synthesized by nucleating and growing nanocrystals on oxidized MWNTs, similar to the synthesis of Ni(OH) 2 on graphene sheets [11] , [14] , [17] . By evaluating pseudocapacitive charge storage of Ni(OH) 2 nanocrystals supported on graphene sheets oxidized to various oxidation degrees, we found that the conductivity of the graphene sheets and their coupling with Ni(OH) 2 nanocrystals were the most important factors in determining the specific capacity and rate capability of the Ni(OH) 2 hybrid materials [14] . Here we employed oxidized MWNTs as novel substrates over graphene sheets for nucleating and growing Ni(OH) 2 nanocrystals. We expect that whereas the functional groups on the oxidized outer walls of the MWNTs could interact with Ni 2+ to initiate nucleation and growth of Ni(OH) 2 nanocrystals, the intact inner walls of the MWNTs could serve as highly conducting wires [18] to provide optimal electrical wiring of the Ni(OH) 2 nanocrystals. The MWNTs used in this work were produced in a fluidized bed reactor that yields ~500 tons of MWNTs annually with high purity (>99.9%) and low cost (material cost ~$10 kg −1 ) [19] , [20] , [21] , [22] . We used a two step solution phase reaction to grow Ni(OH) 2 nanocrystals on oxidized MWNTs ( Supplementary Fig. S1a ), which was also used for the synthesis of various other graphene hybrid nanomaterials by our group [11] , [12] , [14] , [15] , [16] , [17] , [23] . The resulting Ni(OH) 2 /MWNT hybrid contained crystalline β-Ni(OH) 2 nanoplates with irregular shapes interconnected by MWNTs, as revealed by scanning electron microscopy (SEM, Fig. 2a ), transmission electron microscopy (TEM, Fig. 2c,d ) and X-ray diffraction ( Fig. 2b ). The irregular shape of the Ni(OH) 2 nanoplates was an indication of strong interaction of nanoplates with the functional groups and defects on the oxidized MWNTs [11] . Control experiment showed that well defined hexagonal Ni(OH) 2 nanoplates were produced through the same reaction steps without any oxidized MWNTs added ( Supplementary Fig. S2 ). 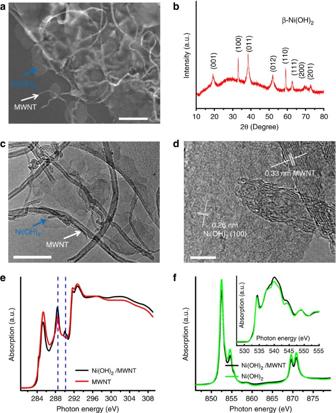Figure 2: Ni(OH)2/MWNT hybrid material. (a) An SEM image of Ni(OH)2nanoplates grown on oxidized MWNTs. Scale bar, 200 nm. (b) X-ray diffraction spectrum of a packed thick film of Ni(OH)2/MWNT. (c) TEM image of Ni(OH)2nanoplates grown on oxidized MWNTs. Scale bar, is 100 nm. (d) A high-resolution TEM image of a Ni(OH)2nanoplate attached to MWNTs. Scale bar, 5 nm. (e) XANES spectra of the Ni(OH)2/MWNT hybrid and the MWNT control sample at carbon K-edge. The blue dashed lines mark the carboxyl π* absorption at 288.5 eV and the carbonate π* absorption at 290.3 eV. (f) XANES spectra of the Ni(OH)2/MWNT hybrid and the Ni(OH)2control sample at nickel L-edge. The inset shows XANES spectra at oxygen K-edge. Figure 2: Ni(OH) 2 /MWNT hybrid material. ( a ) An SEM image of Ni(OH) 2 nanoplates grown on oxidized MWNTs. Scale bar, 200 nm. ( b ) X-ray diffraction spectrum of a packed thick film of Ni(OH) 2 /MWNT. ( c ) TEM image of Ni(OH) 2 nanoplates grown on oxidized MWNTs. Scale bar, is 100 nm. ( d ) A high-resolution TEM image of a Ni(OH) 2 nanoplate attached to MWNTs. Scale bar, 5 nm. ( e ) XANES spectra of the Ni(OH) 2 /MWNT hybrid and the MWNT control sample at carbon K-edge. The blue dashed lines mark the carboxyl π* absorption at 288.5 eV and the carbonate π* absorption at 290.3 eV. ( f ) XANES spectra of the Ni(OH) 2 /MWNT hybrid and the Ni(OH) 2 control sample at nickel L-edge. The inset shows XANES spectra at oxygen K-edge. Full size image X-ray absorption near-edge structure (XANES) measurements were employed to probe the interactions between the Ni(OH) 2 nanoplates and the oxidized MWNTs in the hybrid. The increased absorption intensity at 288.5 eV (carboxyl π*) and 290.3 eV (carbonate π*) at the carbon K-edge of the Ni(OH) 2 /MWNT hybrid (relative to oxidized MWNTs without any metal exposure through the otherwise identical reaction steps) suggested a higher concentration of oxygen functional groups on the MWNT surface bonded with Ni(OH) 2 in the hybrid material ( Fig. 2e ) [24] , [25] . The nickel L-edge absorption confirmed the +2 oxidation state of Ni in both the Ni(OH) 2 /MWNT hybrid and the free Ni(OH) 2 nanoplate sample ( Fig. 2f ). A lower nickel L-edge and a higher oxygen K-edge of the hybrid sample were observed comparing with the free Ni(OH) 2 nanoplate sample, suggesting electron transfer from oxygen to nickel in the hybrid material ( Fig. 2f ) [15] , [26] . The XANES spectroscopic data confirmed strong coupling effects between Ni(OH) 2 nanoplates and oxidized MWNTs in the hybrid. We deposited the Ni(OH) 2 /MWNT hybrid into a Ni foam and investigated the electrochemical properties of the material in 1 M KOH aqueous solution by cyclic voltammetry (CV). The electrode was measured after conditioning and activation steps (see Methods and Supplementary Fig. S3 ). A pair of redox peaks in the voltage range of 0–0.55 V vs saturated calomel electrode (SCE) was observed ( Fig. 3a ) and attributed to the reversible conversion between Ni(II) and Ni(III) [9] , [10] , [14] , [17] . The Ni(OH) 2 nanoplates on MWNTs showed a specific capacity of 228 mAh g −1 and 183 mAh g −1 (based on the mass of Ni(OH) 2 ) at a scan rate of 5 mV s −1 and 40 mV s −1 (corresponding to 13.8 s of a full charging or discharging period, Fig. 3b ) respectively, suggesting excellent rate capability of the hybrid material. The specific capacity ( C s ) was calculated from the CV loops using C s =∫ i / m d t , where i was the oxidation or reduction current, d t was the time differential, and m was the mass of the active electrode material. 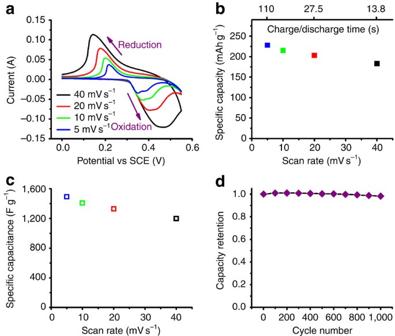Figure 3: Ni(OH)2/MWNT hybrid as a cathode material for the ultra-Ni–Fe battery. (a) CV curves of Ni(OH)2/MWNT hybrid at various scan rates in 1 M KOH. (b) Average specific capacity of Ni(OH)2nanoplates grown on oxidized MWNTs at various scan rates based on CV data in (a). (c) Average specific capacitance within a voltage range of 0.55 V (from 0 V to 0.55 V vs SCE) of Ni(OH)2nanoplates grown on oxidized MWNTs at various scan rates based on CV data in (a). (d) Cycling stability of the Ni(OH)2/MWNT hybrid electrode over 1,000 CV cycles at 100 mV s−1. Loading of Ni(OH)2/MWNT was ~1.1 mg cm−2for the electrode. Figure 3: Ni(OH) 2 /MWNT hybrid as a cathode material for the ultra-Ni–Fe battery. ( a ) CV curves of Ni(OH) 2 /MWNT hybrid at various scan rates in 1 M KOH. ( b ) Average specific capacity of Ni(OH) 2 nanoplates grown on oxidized MWNTs at various scan rates based on CV data in ( a ). ( c ) Average specific capacitance within a voltage range of 0.55 V (from 0 V to 0.55 V vs SCE) of Ni(OH) 2 nanoplates grown on oxidized MWNTs at various scan rates based on CV data in ( a ). ( d ) Cycling stability of the Ni(OH) 2 /MWNT hybrid electrode over 1,000 CV cycles at 100 mV s −1 . Loading of Ni(OH) 2 /MWNT was ~1.1 mg cm −2 for the electrode. Full size image With the ultrafast charging and discharging capability, the Ni(OH) 2 /MWNT hybrid could also be a pseudo-capacitor electrode material when coupled with an electric double layer (EDL) capacitor-like electrode [17] , [27] , [28] . The specific capacitance values of the Ni(OH) 2 nanoplates on MWNTs at various CV scan rates ( Fig. 3c ) were slightly higher than the Ni(OH) 2 nanoplates grown on graphene sheets [14] . The Ni(OH) 2 /MWNT hybrid electrode exhibited high cycling stability with little capacity/capacitance decay over 1,000 cycles ( Fig. 3d ). FeO x /graphene hybrid as anode for ultra-Ni–Fe battery The anode of our ultra-Ni–Fe battery was a FeO x /graphene hybrid, synthesized by a solution phase reaction followed by a gas phase annealing step, similar to our synthesis of a Co 1− x S/graphene hybrid reported previously [13] . In the first step, Fe(OAc) 2 was hydrolyzed in a N , N -dimethylformamide (DMF)/water mixed solvent at 80 °C for coating the GO sheets selectively and uniformly with nanoparticles ( Supplementary Fig. S1b ). In the second step, the intermediate product from the first step was mixed with glucose and annealed in Ar at 550 °C to reduce the GO and make crystalline FeO x particles on graphene. SEM of the FeO x /graphene hybrid ( Fig. 4a ) revealed dense nanoparticle coatings on the reduced GO sheets. X-ray diffraction showed that the FeO x coating on the reduced GO was a mixture of Fe 3 O 4 and metallic Fe ( Fig. 4b ). The Fe 2 p 3/2 electron-binding energy observed in X-ray photoelectron spectroscopy (XPS) spectrum of the FeO x /graphene hybrid was consistent with the X-ray diffraction result, with the peaks at 705 eV and 712 eV corresponding to metallic iron and iron oxide, respectively ( Fig. 4c ). There were two types of particles grown on the graphene sheets, as observed in TEM of the FeO x /graphene hybrid. Most of the particles were in the size range of 5–10 nm ( Fig. 4d,g ), confirmed to be Fe 3 O 4 by selected area electron diffraction ( Fig. 4e ) and high-resolution TEM ( Fig. 4g ). The small sizes of the Fe 3 O 4 nanoparticles were also consistent with broad Fe 3 O 4 peaks in the X-ray diffraction spectrum ( Fig. 4b ). The other type of particles on graphene was metallic iron as evidenced by selected area electron diffraction ( Fig. 4f ). The size of the Fe nanoparticles was about 50–200 nm ( Fig. 4a,d ), giving sharp Fe peaks in the X-ray diffraction spectrum ( Fig. 4b ). On the basis of SEM and TEM observation, only a very small amount (<5%) of iron oxide was reduced to metallic iron presumably by glucose during the annealing step. 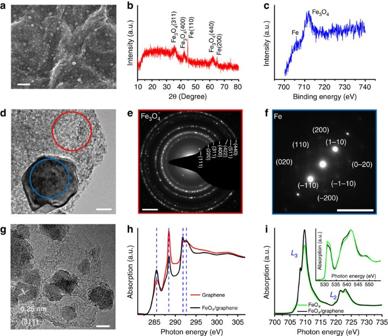Figure 4: FeOx/graphene hybrid material. (a) An SEM image of the FeOx/graphene hybrid. Scale bar, 200 nm. (b) An X-ray diffraction spectrum of a packed thick film of FeOx/graphene. (c) An XPS spectrum of the FeOx/graphene hybrid. (d) A TEM image of FeOx/graphene showing two types of particles grown on graphene. Scale bar, 100 nm. (e) A selected area diffraction pattern of small nanoparticles on graphene in the red circled area of (d). Scale bar, 2 nm−1. (f) A selected area diffraction pattern of a large nanoparticle on graphene in the blue circled area of (d). Scale bar, 10 nm−1. (g) High-resolution TEM image of small Fe3O4nanoparticles grown on graphene. Scale bar, 5 nm. (h) XANES spectra of the FeOx/graphene hybrid and the graphene control sample at carbon K-edge. Blue dashed lines mark the graphene π* absorption at 285.5 eV, carboxyl π* absorption at 288.5 eV, and graphene σ* absorption at 291.8 and 292.7 eV. (i) XANES spectra of the FeOx/graphene hybrid and the FeOxcontrol sample at iron L-edge. The inset shows XANES spectra at oxygen K-edge. Figure 4: FeO x /graphene hybrid material. ( a ) An SEM image of the FeO x /graphene hybrid. Scale bar, 200 nm. ( b ) An X-ray diffraction spectrum of a packed thick film of FeO x /graphene. ( c ) An XPS spectrum of the FeO x /graphene hybrid. ( d ) A TEM image of FeO x /graphene showing two types of particles grown on graphene. Scale bar, 100 nm. ( e ) A selected area diffraction pattern of small nanoparticles on graphene in the red circled area of ( d ). Scale bar, 2 nm −1 . ( f ) A selected area diffraction pattern of a large nanoparticle on graphene in the blue circled area of ( d ). Scale bar, 10 nm −1 . ( g ) High-resolution TEM image of small Fe 3 O 4 nanoparticles grown on graphene. Scale bar, 5 nm. ( h ) XANES spectra of the FeO x /graphene hybrid and the graphene control sample at carbon K-edge. Blue dashed lines mark the graphene π* absorption at 285.5 eV, carboxyl π* absorption at 288.5 eV, and graphene σ* absorption at 291.8 and 292.7 eV. ( i ) XANES spectra of the FeO x /graphene hybrid and the FeO x control sample at iron L-edge. The inset shows XANES spectra at oxygen K-edge. Full size image The FeO x /graphene electrode was prepared by mixing the intermediate product from the first step reaction with glucose and polytetrafluoroethylene (PTFE), depositing into Ni foam, and then annealing in Ar at 550 °C (see Methods ). It was important to load the material into Ni foam before high temperature annealing to afford hybrid materials uniformly dispersed and adhered to the Ni foam. The addition of glucose during this step was found to improve the stability of the resulting hybrid for electrochemical cycling. The electrochemical characteristics of the FeO x /graphene electrode were investigated in 1 M KOH solutions. Multiple peaks showed up in the first several CV cycles, corresponding to various redox reactions of iron species with different oxidation states ( Supplementary Fig. S4 ) [29] , [30] , [31] . After ~20 conditioning cycles, the CV curve stabilized with only one pair of redox peaks remaining ( Fig. 5a ), corresponding to conversion between Fe(II) and Fe(0) [9] , [10] , [29] , [30] , [31] . When scanned to the more negative potential direction, Fe(II) was reduced to Fe(0) before appreciable hydrogen evolution ( Fig. 5a ). Fe(0) was oxidized to Fe(II) when scanned to the positive direction, consistent with the single oxidation peak observed in CV ( Fig. 5a ). The FeO x nanoparticles grown on graphene exhibited a specific capacity of 377 mAh g −1 based on the FeO x mass at a scan rate of 5 mV s −1 ( Fig. 5b ), corresponding to a specific pseudo-capacitance of 1,131 F g −1 within a voltage range of 1.2 V ( Fig. 5c ). At a high scan rate of 40 mV s −1 , which corresponded to a full charging or discharging time of 27.5 s, the capacity was still as high as 317 mAh g −1 ( Fig. 5b ). After the conditioning CV scans, no large Fe particles were observed in the TEM ( Supplementary Fig. S5 ), indicating the initial Fe particles were electrochemically active and broke into small ones during the conditioning cycles. The steady redox peaks of the FeO x /graphene hybrid were in the range of −0.5 V to −1.3 V vs SCE, making it a suitable electrode to pair with the Ni(OH) 2 /MWNT hybrid to form a battery. 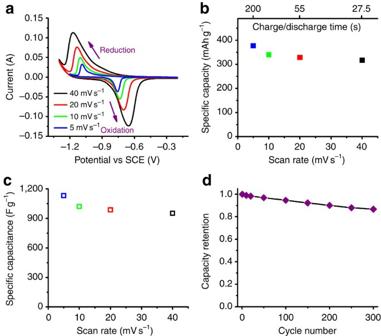Figure 5: FeOx/graphene hybrid as an anode material for the ultra-Ni–Fe battery. (a) CV curves of FeOx/graphene hybrid at various scan rates in 1 M KOH. (b) Average specific capacity of FeOxnanoparticles grown on graphene at various scan rates based on CV data in (a). (c) Average specific capacitance within a voltage range of 1.2 V (from −0.2 V to −1.4 V vs SCE) of FeOxnanoparticles grown on graphene at various scan rates based on CV data in (a). (d) Cycling stability of the FeOx/graphene hybrid over 300 CV cycles at 40 mV s−1. Loading of FeOx/graphene was ~0.7 mg cm−2for the electrode. Figure 5: FeO x /graphene hybrid as an anode material for the ultra-Ni–Fe battery. ( a ) CV curves of FeO x /graphene hybrid at various scan rates in 1 M KOH. ( b ) Average specific capacity of FeO x nanoparticles grown on graphene at various scan rates based on CV data in ( a ). ( c ) Average specific capacitance within a voltage range of 1.2 V (from −0.2 V to −1.4 V vs SCE) of FeO x nanoparticles grown on graphene at various scan rates based on CV data in ( a ). ( d ) Cycling stability of the FeO x /graphene hybrid over 300 CV cycles at 40 mV s −1 . Loading of FeO x /graphene was ~0.7 mg cm −2 for the electrode. Full size image We found that the cycling stability of the FeO x /graphene hybrid electrode was strongly affected by parameters such as KOH concentration of the electrolyte, Fe/C ratio of the hybrid, glucose additive, and annealing temperature ( Supplementary Fig. S6 ). In particular, glucose addition to the FeO x /graphene hybrid material followed by thermal annealing improved cycling stability by mitigating aggregation of the FeO x nanoparticles. SEM imaging revealed that without glucose addition, large (~200–500 nm) rod-like structures were formed in the electrode material after 300 CV cycles in 1 M KOH ( Supplementary Figs S7a and S7b ). In contrast, with glucose addition, a much lesser degree of aggregation was observed, with most of the FeO x remaining as nanoparticles on the graphene sheets ( Supplementary Figs S7c and S7d ). This might be owing to a thin layer of carbon coating formed on the FeO x nanoparticles through glucose decomposition, impeding the nanoparticles from aggregation during cycling. We used another carbon precursor, 10,10-dibromo-9,9-bianthryl to replace glucose and obtained a FeO x /graphene material with comparable cycling stability as the glucose-treated one. Even with all the above parameters optimized, a discernible decay in capacity/capacitance was still observed for the FeO x /graphene electrode over hundreds of CV cycles ( Fig. 5d ). This instability could be associated with the eventual aggregation of FeO x nanoparticles through many reaction cycles, as revealed by SEM imaging of the electrode material after more than 1,000 electrochemical cycles ( Supplementary Fig. S8 ). Aggregation of the FeO x nanoparticles indicated the loss of nanoparticle bonding and coupling with the conducting graphene sheets, leading to reduced electrochemical activity. To understand the excellent electrochemical capacity and rate performance of the FeO x /graphene hybrid, we performed XANES measurements to investigate the interactions between FeO x nanoparticles and graphene in the hybrid. To avoid interference with the carbon signal from graphene, no glucose was added in the annealing step of the sample prepared for XANES. At the carbon K-edge ( Fig.4h ), the FeO x /graphene hybrid showed a clear increase in absorption intensity at 285.5 eV compared with a control-reduced GO sample that had gone through the same synthesis and processing steps as the hybrid except for without adding any Fe(OAc) 2 . This increased absorption suggested a higher π* density and thus enhanced sp 2 bonding characteristics [24] . This was consistent with the better resolved resonances, at 291.8 and 292.7 eV, that indicated a more restored graphitic lattice in the hybrid [24] . The absorption peak at 288.5 eV (carboxyl π*) near the carbon K-edge was attributed to C–O functional groups in the reduced GO and could be affected by covalent Fe–O–C bonding [24] , [25] . At the iron L-edge XANES ( Fig. 4i ), the L 3 and L 2 peaks were consistent with the Fe 3 O 4 phase [32] , [33] . The increased iron L-edge and the decreased oxygen K-edge ( Fig. 4i inset) of the hybrid compared with the free FeO x control suggested an increase in the unoccupied electron density states at the O site and a decrease in the unoccupied electron density states at the Fe site, consequently a higher ionic Fe-O bonding in the hybrid [15] , [26] . Ultra-Ni–Fe battery made of Ni(OH) 2 /MWNT and FeO x /graphene A two-electrode ultra-Ni–Fe cell was fabricated by using the Ni(OH) 2 /MWNT hybrid material as the cathode and the FeO x /graphene hybrid material as the anode in 1 M KOH ( Fig. 6a , 1.1 mg of Ni(OH) 2 /MWNT and 0.7 mg of FeO x /graphene were loaded into 1 cm 2 Ni foams to form the electrodes). The mass ratio of Ni(OH) 2 /FeO x was chosen to balance the cathode capacity with the anode capacity. CV curves of the ultra-Ni–Fe cell at various scan rates corresponding to a full charging or discharging time from ~20 s to ~3 min are shown in Fig. 6a . At such high charging and discharging rates, the ultra-Ni–Fe cell was able to achieve high specific capacity from 102 mAh g −1 to 125 mAh g −1 based on total mass of the active materials ( Fig. 6b ), confirming the exceptional rate capability of the hybrid nanomaterials. 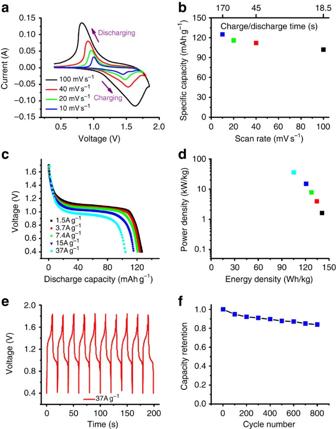Figure 6: Ultra-Ni–Fe battery made of Ni(OH)2/MWNT and FeOx/graphene. (a) CV curves at various scan rates in two-electrode configuration in 1 M KOH. 1.1 mg of Ni(OH)2/MWNT and 0.7 mg of FeOx/graphene were loaded into 1 cm2Ni foams to form the electrodes. (b) Two-electrode specific capacity of the ultra-Ni–Fe battery at various scan rates based on CV data in (a). (c) Galvanostatic discharge curves at various current densities. Charging was performed at 3.7 A g−1till 1.67 V. (d) Ragone plot of the ultra-Ni–Fe battery measured in (c). (e) Galvanostatic charge and discharge curves of the ultra-Ni–Fe at a current density of 37 A g−1. (f) Capacity retention vs cycle number for the ultra-Ni–Fe battery at a galvanostatic charge and discharge current density of 37 A g−1. Figure 6: Ultra-Ni–Fe battery made of Ni(OH) 2 /MWNT and FeO x /graphene. ( a ) CV curves at various scan rates in two-electrode configuration in 1 M KOH. 1.1 mg of Ni(OH) 2 /MWNT and 0.7 mg of FeO x /graphene were loaded into 1 cm 2 Ni foams to form the electrodes. ( b ) Two-electrode specific capacity of the ultra-Ni–Fe battery at various scan rates based on CV data in ( a ). ( c ) Galvanostatic discharge curves at various current densities. Charging was performed at 3.7 A g −1 till 1.67 V. ( d ) Ragone plot of the ultra-Ni–Fe battery measured in ( c ). ( e ) Galvanostatic charge and discharge curves of the ultra-Ni–Fe at a current density of 37 A g −1 . ( f ) Capacity retention vs cycle number for the ultra-Ni–Fe battery at a galvanostatic charge and discharge current density of 37 A g −1 . Full size image The ultra-Ni–Fe cell performance was further evaluated by galvanostatic measurements. Figure 6c shows discharging voltage profiles of the ultra-Ni–Fe cell at various current densities. Charging was performed at a current density of 3.7 A g −1 . To calculate the specific capacity, we used the equation C s = I Δ t / m , where I was the discharging current, Δ t was discharging time, and m was the total mass of the active electrode materials. At high discharging current densities from 1.5 A g −1 to 37 A g −1 , our ultra-Ni–Fe cell was able to deliver specific capacity ranging from 126 mAh g −1 to 104 mAh g −1 ( Fig. 6c ), based on the total mass of the active materials. This was consistent with the capacity values measured by CV ( Fig. 6b ). Discharge at various rates as shown in Fig. 6c was completed in from ~5 min to ~9 s, and charging was completed in about 2 min, much faster than conventional Ni–Fe batteries that need to be charged and discharged in hours [9] , [10] . Our battery also outperformed a recently reported Ni–Fe battery (made from Fe 2 O 3 nanorods supported on carbon nanofibres and β-Ni(OH) 2 ) with a specific capacity of ~80 mAh g −1 (based on active material mass) and hour-scale charging and discharging times [34] . Thus, the ultra-Fe–Ni battery made of strongly coupled hybrid materials afforded unprecedented high-rate performance of rechargeable batteries in an aqueous electrolyte. The average discharge voltages of our ultra-Ni–Fe cell shown in Fig. 6c were from ~1.1 V to ~0.95 V, making it a feasible cell for energy storage. The energy and power densities ( d e and d p ) were calculated for the ultra-Ni–Fe cell and shown in the Ragone plot in Fig. 6d , using equations and d p = d e /Δ t , where I was the discharging current, V was discharging voltage, d t was time differential, m was the total mass of the active electrode materials, and Δ t was the discharging time. Our ultra-Ni–Fe cell showed an energy density of 141 Wh kg −1 at a power density of 1.6 kW kg −1 , and a power density of 36 kW kg −1 at an energy density of 105 Wh kg −1 . This suggested nearly 1,000-fold increase of the power rate of Ni–Fe batteries without losing energy capacity. Cycle life of the ultra-Ni–Fe cell was measured by galvanostatic measurements at a current density of 37 A g −1 ( Fig. 6e ). Coulombic efficiency was near 100% during the ultrafast cycling ( Fig. 6e ). About ~80% of the initial capacity was maintained after 800 cycles of charge–discharge ( Fig. 6f ). The capacity decay was most likely due to the FeO x /graphene electrode rather than the Ni(OH) 2 /MWNT electrode, which could be deduced from the half-cell performances of the two electrodes ( Figs 5d and 3d ) [34] . Even faster capacity decay was observed in a recent Ni–Fe battery made from Fe 2 O 3 nanorods supported on carbon nanofibres and β-Ni(OH) 2 (~8% decay for 100 cycles) [34] . Further work is needed to further understand and eliminate the decay of the FeO x /graphene anode. Nevertheless, because of the low cost, high safety and environmentally friendliness, the ultra-Ni–Fe battery with ultrafast charge and discharge at high energy density holds promise for power quality applications ranging from portable electronics, emergency power supply, transportation, and electrical grid. With increased mass loading of electrode materials (1.9–3.0 mg cm −2 for Ni(OH) 2 /MWNT and 1.4–2.1 mg cm −2 for FeO x /graphene), specific capacity in the range of ~105–125 mAh g −1 was obtained for the ultra-Ni–Fe battery ( Supplementary Fig. S9 ), compared with ~125 mAh g −1 at 1.1 mg cm −2 of Ni(OH) 2 /MWNT and 0.7 mg cm −2 of FeO x /graphene ( Fig. 6 ). We compared our ultra-Ni–Fe cell with an EDL supercapacitor made up of high performance activated carbon (~300 F g −1 at ~1 mg cm −2 ) in the same KOH aqueous electrolyte ( Supplementary Fig. S10 ). With ~5-fold lower active material mass, the ultra-Ni–Fe cell provided ~2-fold higher energy and power than the EDL supercapacitor with mass loading of ~10 mg cm −2 ( Supplementary Figs S11a and S11c ), suggesting the ultra-Ni–Fe battery with more than an order of magnitude higher specific energy and power ( Supplementary Figs S11b and S11d ) than typical supercapacitors in aqueous electrolytes. The superior performance of the ultra-Ni–Fe cell is attributed to the unique structures of the inorganic/carbon hybrid materials. The Ni(OH) 2 nanoplates and FeO x nanoparticles are directly and selectively grown on the nanocarbon substrates. The bonding and coupling between the nano-sized active materials and nanocarbon in the hybrid structures drastically enhance charge transfer in the electrodes. In a control experiment, we synthesized free Ni(OH) 2 nanoplates and FeO x nanoparticles following the same procedures as for the hybrid materials but without any nanocarbon added. Their mixtures with carbon black showed much lower specific capacities than the hybrid materials ( Supplementary Fig. S12 ). This clearly demonstrates the advantage of our inorganic/carbon hybrid materials. In summary, we have synthesized new Ni(OH) 2 /MWNT and FeO x /graphene hybrid materials with excellent electrochemical performances by utilizing the high conductivity of the graphitic carbon materials and strong coupling between inorganic nanocrystals and oxidized nanocarbon. Pairing of the two hybrid materials affords an ultrafast version of Ni–Fe battery capable of charge and discharge in seconds. With comparable energy density as conventional Ni–Fe batteries, the new ultra-Ni–Fe battery achieves nearly 1,000 times higher power density, making it a high-performance, low cost, safe and environmentally benign energy storage device. Making of GO and oxidized MWNTs GO was made by a modified Hummers method. Graphite flakes (1 g, Superior Graphite) were ground with NaCl (~10 g) for 10 min. Afterwards, NaCl was washed away by repeatedly rinsing with water in a vacuum filtration apparatus. The remaining graphite was heated at 70 °C in an oven for 20 min to remove the remaining water. The dried solid was then combined with 23 ml of concentrated sulphuric acid in a 250 ml round bottom flask and stirred at room temperature for 24 h. Next, the flask was placed in an oil bath at 40 °C and 100 mg of NaNO 3 was added to the suspension and allowed to be dissolved for 5 min. This step was followed by the slow addition of 500 mg (3 g for the Hummers GO) of KMnO 4 , keeping the temperature below 45 °C. The solution was allowed to stir for 30 min. Afterwards, 3 ml of water was added to the flask, followed by another 3 ml after 5 min. In another 5 min, 40 ml of water was added. After 15 min, the solution was removed from the oil bath and 140 ml of water and 10 ml of 30% H 2 O 2 were added to end the reaction. This suspension was stirred at room temperature for 5 min. The suspension was then repeatedly centrifuged and washed twice with 5% HCl solution and then repeatedly with water. The collected precipitate was dispersed in 150 ml of anhydrous DMF and cup-horn sonicated for 20 min. After 5,000 r.p.m. centrifuge (3,020 g ) for 5 min, a dark brown homogeneous supernatant was obtained. Oxidized MWNTs were made by a modified Hummers method. MWNTs (1 g, FloTube 9000 from CNano Technology) were first purified by calcination at 500 °C for 1 h and washing with diluted hydrochloric acid (10%). The purified MWNTs were put into a 250 ml round-bottom flask. 23 ml of concentrated sulphuric acid was added and the mixture was stirred at room temperature overnight. Next, the flask was heated in an oil bath at 40 °C and 350 mg of NaNO 3 was added to the suspension and allowed to be dissolved for 5 min. This step was followed by the slow addition of 2 g of KMnO 4 , keeping the reaction temperature below 45 °C. The solution was stirred for 30 min. Afterwards 3 ml of water was added to the flask, followed by another 3 ml after 5 min. After another 5 min, 40 ml of water was added. 15 min later, the flask was removed from the oil bath and 140 ml of water and 10 ml of 30% H 2 O 2 were added to end the reaction. This suspension was stirred at room temperature for 5 min. It was then repeatedly centrifuged and washed with 5% HCl solution twice, followed by rinsing with copious amounts of water. The final precipitate was dispersed in 10 ml of water and lyophilized. Finally, a dry product of ~1 g was collected. Synthesis of Ni(OH) 2 /MWNT hybrid and FeO x /graphene hybrid In a typical synthesis of Ni(OH) 2 /MWNT hybrid, ~4 mg of oxidized MWNTs were dispersed in 8 ml of anhydrous DMF, to which 0.8 ml of 0.2 M Ni(OAc) 2 aqueous solution was added. The suspension was kept at 80 °C with magnetic stirring for 4 h. After that, the intermediate product was collected by centrifuge and washing with water. The intermediate product was then dispersed in ~12 ml of water. The suspension was then sealed in a 40-ml Teflon-lined stainless steel autoclave for hydrothermal reaction at 180 °C for 12 h. The final product was collected by centrifuge, water-washing and lyophilization. To synthesize the FeO x /graphene hybrid, 0.8 ml of 0.2 M Fe(OAc) 2 aqueous solution was added to 8 ml of GO DMF suspension (~0.3 mg ml −1 ). The suspension was kept at 80 °C with magnetic stirring for 2 h. After that, the intermediate product was collected by centrifugation, washed with water, and lyophilized. The intermediate product was then mixed with glucose and annealed in Ar at 550 °C for 1 h to produce the final FeO x /graphene hybrid (To prepare the FeO x /graphene electrode with optimal dispersion of the hybrid material, the material was first loaded into Ni foam and then annealed; see below). There was a mass loss of ~40% associated with this step, owing to evaporation of adsorbed and hydrated water in the material. The mass ratios of nanocarbon in the hybrid materials were determined by thermal gravimetric experiments, in which the hybrid materials were heated in air at 500 °C for 3 h. The MWNTs and graphene were burned away and Ni(OH) 2 and FeO x were transformed to NiO and Fe 2 O 3 , respectively. The mass ratios of nanocarbon were then calculated accordingly, based on the mass loss of the materials. We found that the Ni(OH) 2 /MWNT hybrid contained ~30% of MWNTs by mass and the FeO x /graphene hybrid contained ~20% of graphene by mass. Characterization SEM was carried out on an FEI XL30 Sirion scanning electron microscope. TEM was carried out on an FEI Tecnai G2 F20 transmission electron microscope. X-ray diffraction was carried out on a PANalytical X'Pert instrument. XPS measurement was performed on an SSI S-Probe XPS Spectrometer. XANES data were recorded in the surface-sensitive total electron yield with the use of specimen current. Data were first normalized to the incident photon flux I 0 measured with a refreshed gold mesh at SGM before the measurement. After background correction, the XANES are then normalized to the edge jump, the difference in absorption coefficient just below and at a flat region above the edge. CV and chronopotentiometry were carried out on a CHI 760D electrochemistry workstation. Preparation of working electrodes To prepare the Ni(OH) 2 /MWNT electrode, Ni(OH) 2 /MWNT hybrid material was first mixed with PTFE (from 60wt.%. water suspension, Aldrich) in a ratio of 100:2 by weight, and then dispersed in ethanol; the suspension was drop-dried into a 1 cm×1 cm Ni foam (2-mm thick, 100 ppi, 95% porosity, Marketech) at 80 °C; the electrode was then baked at 120 °C for 20 min; the electrode was compressed to ~0.5 mm thick before measurement. To prepare the FeO x /graphene hybrid electrode, the intermediate product after the first-step reaction at 80 °C was first mixed with glucose and PTFE in a ratio of 100:20:5 by weight, and then dispersed in ethanol; the suspension was drop-dried into a 1 cm×1 cm Ni foam at 80 °C. The electrode was then annealed in 1 Torr Ar at 550 °C for 1 h; the annealed electrode was compressed to ~0.5 mm thickness before measurement. All the working electrodes in this work were prepared following the above procedures unless otherwise noted. Electrodes of free Ni(OH) 2 and FeO x mixed with carbon black were prepared in the same way as the hybrid electrodes except that mixtures were used to replace the hybrid materials. To prepare the activated carbon electrode, activated carbon was mixed with carbon black and polyvinylidene difluoride in a ratio of 10:1:1 in N -methyl-2-pyrrolidone by magnetic stirring for 12 h. The mixture was then pasted onto Ni foam, dried at 80 °C and further baked at 200 °C for 1 h in air. Mass loadings for the pasted electrodes were determined by comparing the mass of the electrode with that of the original blank Ni foam. Electrochemical measurements Electrochemical measurements were carried out in a beaker cell with 1 M KOH aqueous solution as the electrolyte. CV measurements of the Ni(OH) 2 /MWNT and FeO x /graphene electrodes were performed in a three-electrode configuration, where a SCE was used as the reference electrode, and a graphite rod was used as the counter electrode. Conditioning and activation steps were applied to the Ni(OH) 2 /MWNT electrode before electrochemical data were taken. 200 conditioning CV scans at 40 mV s −1 were first performed, and then the electrode was dried without rinsing off the electrolyte solution and kept in ambient conditions for 3–10 days for activation. We found electrodes with higher mass loadings of the Ni(OH) 2 /MWNT material took longer to be activated. Blank Ni foam that went through the same conditioning and activation steps as the Ni(OH) 2 /MWNT hybrid electrode showed negligible capacity compared with the hybrid electrode ( Supplementary Fig. S3 ). The activation step was not effective for the blank Ni foam ( Supplementary Fig. S3 ). The Ni–Fe battery was measured in a two-electrode configuration, where the reference lead was connected to the counter electrode lead. The Ni(OH) 2 /MWNT electrode was pre-scanned against the reference electrode at 40 mV s −1 for 200 cycles and left dried with KOH solution inside for 3–10 days to stabilize the capacitance/capacity before further measurements. The FeO x /graphene electrode was pre-scanned against the reference electrode at 100 mV s −1 for 20 cycles to stabilize the capacitance/capacity before further measurements. For all the electrodes, we performed experiments to make sure that the capacitance contribution from the Ni foam was negligible. How to cite this article: Wang, H. et al . An ultrafast nickel–iron battery from strongly coupled inorganic nanoparticle/nanocarbon hybrid materials. Nat. Commun. 3:917 doi: 10.1038/ncomms1921 (2012).